Past daily light cycle recorded in the strontium/calcium ratios of giant clam shells The historical record of daily light cycle in tropical and subtropical regions is short. Moreover, it remains difficult to extract this cycle in the past from natural archives such as biogenic marine carbonates. Here we describe the precise analysis of Sr/Ca, Mg/Ca, and Ba/Ca ratios in a cultivated giant clam shell, using a laterally high-resolution secondary ion mass spectrometer with 2 μm resolution. The Sr/Ca ratio exhibits striking diurnal variations, reflecting the daily light cycle. A clear seasonal variation in Sr/Ca is also observed in another longer set of measurements with 50 μm resolution. Light-enhanced calcification and elemental transportation processes, in giant clam and symbiotic algae, may explain these diurnal and annual variations. This opens the possibility to develop the Sr/Ca ratio from a giant clam shell as an effective proxy for parameters of the daily light cycle. In tropical and subtropical regions, instrumental records as well as historical documents are relatively short compared with those in the temperate zones. Also, dendroclimatology is difficult to apply in low latitudes. Thus, biogenic marine carbonates are important tools for reconstruction of the past climate system. Proxies reflecting past seawater temperature [1] , [2] , [3] , salinity [4] , [5] , pH [6] , [7] , and nutrients [8] , [9] has been derived from stable isotopes and trace elements in coral skeletons, foraminifera tests, and mollusk shells. Insolation is an important component of meteorological data, as solar energy is the primal and direct driver of weather and climate. Proxy development for reconstruction of light cycle can open new opportunities on past climate study; in that, the insolation is a 'driving force' whereas conventional proxies reconstruct the consequential 'environment'. Few attempts have been made to estimate the past light cycle with hourly insolation, using environmental proxies such as carbonate chemistry and isotopes [10] , [11] , but none has succeeded. Several recent microanalytical studies have extracted valuable knowledge related to palaeoclimate data [12] , [13] , but not the daily light cycle. In this study, we analysed strontium/calcium of giant clam shells with a 2-μm resolution using laterally high-resolution secondary ion mass spectrometry. We observe synchronous, daily variations in Sr/Ca and growth-banding pattern, pointing to the possibility of reconstructing daily light cycle at a few hour timescale. This is the finest spatial resolution in the literature of carbonate geochemistry. Sample description and Sr/Ca imaging Live giant clams ( Tridacna derasa ) were collected from Kabira coral reef at Ishigaki Island (124°09′ E, 24°20′ N) in the southwestern part of the Ryukyu Archipelago, southern Japan, on October 14, 2005. Kabira is a well-developed fringing coral reef with a typical zonation from land to ocean including a moat, inner reef flat, reef crest, outer reef flat, and reef slope. The sampled T. derasa had been cultivated in the reef since 27 March 2002, and environmental data such as precipitation, temperature, insolation, sea level, and seawater temperature were measured automatically in the reef and documented until the collection date. After removing the soft tissue, the centre of one side of the shell was cut from its umbo to the ventral margin along the maximum growth axis ( Fig. 1a ). Then a radial section was prepared using a dental cutting machine ( Fig. 1b ). An inner layer part was mounted in epoxy resin disk together with a carbonate standard ( Fig. 1c ). This species is known to form a growth line each day [14] , [15] , [16] , and to facilate age-model determination by counting growth lines, Sr enrichment band was measured using an electron probe microanalyzer (EPMA; Fig. 1d,e ). On cloudy or rainy days, there were probably irregular Sr bands for the day, which can be corrected to assign calendar date (Methods). 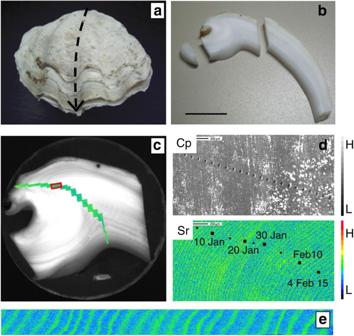Figure 1: Photograph of cutting section and strontium imaging of giant clam shell. (a) Photograph ofT. deraracultivated at Ishigaki Island in the southwestern part of Ryukyu Archipelago, southern Japan. A dotted arrow indicates the vertical cutting section of the half-valve. (b) Section of the half-valve. The black bar shown at the bottom denotes a 2-cm scale bar. (c) Photograph of the cutting section obtained using a commercial photo scanner anlaysed in this work together with small figures obtained using an EPMA. The trajectory of the figures coincides with that of SIMS analysis. (d) Composite image (Cp) and Sr concentration map (Sr) of the sample enlarged from a red square marked in (c). Dates were counted using the daily growth lines with Sr enrichment bands. (e) Enlarged image of Sr concentration map of another region measured using an EPMA. The high and low Sr contents show thin and thick bands. Figure 1: Photograph of cutting section and strontium imaging of giant clam shell. ( a ) Photograph of T. derara cultivated at Ishigaki Island in the southwestern part of Ryukyu Archipelago, southern Japan. A dotted arrow indicates the vertical cutting section of the half-valve. ( b ) Section of the half-valve. The black bar shown at the bottom denotes a 2-cm scale bar. ( c ) Photograph of the cutting section obtained using a commercial photo scanner anlaysed in this work together with small figures obtained using an EPMA. The trajectory of the figures coincides with that of SIMS analysis. ( d ) Composite image (Cp) and Sr concentration map (Sr) of the sample enlarged from a red square marked in ( c ). Dates were counted using the daily growth lines with Sr enrichment bands. ( e ) Enlarged image of Sr concentration map of another region measured using an EPMA. The high and low Sr contents show thin and thick bands. Full size image High-resolution profiles Four sets of trace element profiles for Sr/Ca, Mg/Ca, and Ba/Ca ratios from two individual T. derasa were obtained using a laterally high-resolution secondary ion mass spectrometer [17] , (NanoSIMS) along the growth axis of the juvenile clam shell. In the first, 'high'-resolution set measurements were made along the growth axis with a 2-μm spot at 2 μm interval from the inner edge ( Fig. 1c ). The edge was last calcified and is thus expected to correspond to the sample collection date. The error in the Sr/Ca measurement is about 2% (1 σ ) as estimated by repeated measurements of a standard calcite. Because the collection time is known, it is possible to determine the calendar dates for this record by counting growth layers from the inner edge. The Sr/Ca ratio varies regularly and indicates a clear diurnal signal ( Fig. 2a ), suggesting that environmental parameters such as solar radiation and/or temperature drive the giant clam shell Sr/Ca geochemistry. The conclusion that the Sr/Ca ratio reflects the diurnal signal is robust and significant, because the Sr/Ca variability shown in Fig. 2a is reproduced in the second set of high-resolution measurements obtained from a different T. derasa individual living at the same location during the same time period ( Supplementary Fig. S1 ). Interestingly, the number of data representing a single day is approximately twice in the first record shown in Fig. 2 than in the second record. As both data sets had the same 2-μm sampling resolution, the daily bandwidth is different by a factor of two, indicating that the growth rate can be quite variable among the individuals living under presumably the same environmental conditions. 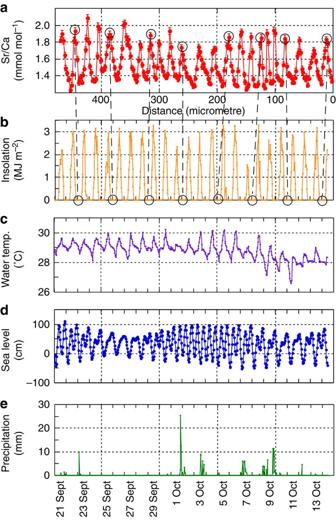Figure 2: High-resolution profile of Sr/Ca ratio in giant clam shell with environmental data. (a) Diurnal variation of Sr/Ca in the giant clam shell as a function of distance from the inner shell edge. The distance was imposed to match the date of meteorological data by a counting of daily growth lines. Error assigned to the symbol is 1σ. (b) Record of insolation during the time interval of Sr/Ca observation at Ishigaki Island. (c) Surface seawater temperatures at Shiraho coral reef, close to Kabira, at the island where the giant clam was cultivated. (d) Record of sea level at Shraho coral reef. (e) Precipitation record at Ishigaki Island. Figure 2: High-resolution profile of Sr/Ca ratio in giant clam shell with environmental data. ( a ) Diurnal variation of Sr/Ca in the giant clam shell as a function of distance from the inner shell edge. The distance was imposed to match the date of meteorological data by a counting of daily growth lines. Error assigned to the symbol is 1 σ . ( b ) Record of insolation during the time interval of Sr/Ca observation at Ishigaki Island. ( c ) Surface seawater temperatures at Shiraho coral reef, close to Kabira, at the island where the giant clam was cultivated. ( d ) Record of sea level at Shraho coral reef. ( e ) Precipitation record at Ishigaki Island. Full size image Low-resolution profiles The third and longest set of new Sr/Ca data, which is referred to here as the 'low'-resolution record, spans 2 years of growth ( Fig. 3 ). Measurements were made with 10-μm diameter spots at 50 μm interval along the same growth line in the same bivalve sample, from which the high-resolution data were obtained. The annual variation of Sr/Ca ratios, low in summer and high in winter, is clearly visible. This general trend is observable and confirmed by ICP-MS measurements ( Supplementary Fig. S2 ). The analytical error of the Sr/Ca ratio in this long record is again ~2% (1 σ ). The age model for this record was guided by our preliminary conclusion that calcification rate is faster, and growth band is wider during the day than night (see Discussion and Methods for more details of the age model and the fourth data set, which presents four short segments of the long record at select intervals at high resolution). 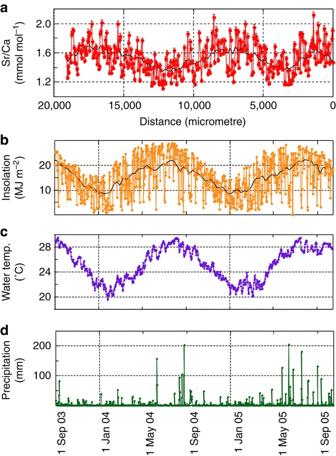Figure 3: Low-resolution profile of Sr/Ca ratio in giant clam shell with environmental data. (a) Annual variation of Sr/Ca ratios in the giant clam shell as a function of distance from the inner shell edge. The distance was imposed to match the date of meteorological data by counting of daily growth lines. Error assigned to the symbol is 1σ. (b) Record of insolation during the possible time interval of Sr/Ca observation at Ishigaki Island. (c) Surface seawater temperature in the Kabira coral reef at the island where the giant clam was cultivated. (d) Precipitation record at Ishigaki Island. Figure 3: Low-resolution profile of Sr/Ca ratio in giant clam shell with environmental data. ( a ) Annual variation of Sr/Ca ratios in the giant clam shell as a function of distance from the inner shell edge. The distance was imposed to match the date of meteorological data by counting of daily growth lines. Error assigned to the symbol is 1 σ . ( b ) Record of insolation during the possible time interval of Sr/Ca observation at Ishigaki Island. ( c ) Surface seawater temperature in the Kabira coral reef at the island where the giant clam was cultivated. ( d ) Precipitation record at Ishigaki Island. Full size image As a result of how the age model was constructed and because insolation variation leads water temperature variation, the low-resolution Sr/Ca record also has a negative correlation with monthly mean insolation, but not with monthly mean water temperature ( Fig. 3 ; Supplementary Fig. S3 ). We note that a previous study, which measured Sr/Ca in a different bivalve species Tridacna gigas, showed no clearly reproducible seasonal trend [18] . The discrepancy with this work may be attributable to the coarser analytical spatial resolution (70-μm spot diameter by laser ablation ICP-MS), or to the particular age of the clam individual used in the previous study. The associated low-resolution Mg/Ca and Ba/Ca measurements ( Supplementary Fig. S4 ) show features similar to the same measurements made in the high-resolution record ( Fig. 4 ). Namely, both Mg/Ca and Ba/Ca records are spiker than Sr/Ca, and Ba/Ca show no obvious correlation to Sr/Ca. 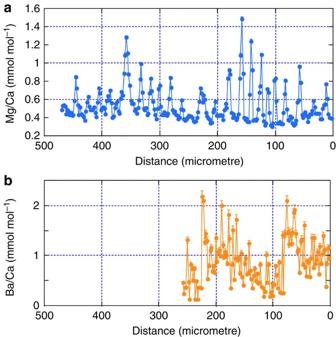Figure 4: High-resolution profiles of Mg/Ca and Ba/Ca ratios in giant clam shell. (a) Mg/Ca ratios and (b) Ba/Ca ratios, as a function of distance from the inner shell edge. These data correspond to the Sr/Ca data inFig. 2a. Ba/Ca data between 250 and 470 μm are lacking because of unexpected instability of the deflector plate located just before the ion-counting detector for138Ba ions. Figure 4: High-resolution profiles of Mg/Ca and Ba/Ca ratios in giant clam shell. ( a ) Mg/Ca ratios and ( b ) Ba/Ca ratios, as a function of distance from the inner shell edge. These data correspond to the Sr/Ca data in Fig. 2a . Ba/Ca data between 250 and 470 μm are lacking because of unexpected instability of the deflector plate located just before the ion-counting detector for 138 Ba ions. Full size image In this study, layer counting does not allow definitive determination of how Sr/Ca varies with time, as the growth rate is not known and probably varies with time. Specifically, it is unclear a priori which parts of the diurnal Sr/Ca variation correspond to day and night. In Fig. 2a , Sr/Ca peaks generally consist of few data points, whereas the troughs consist of a larger number of data. The peaks are thus narrower than the troughs, and this is consistent with the alternating bandwidths of the Sr concentration map ( Fig. 1e ). Because photosynthetic activity of symbiotic dinoflagellates, and, hence, the clam shell calcification rate are expected to be enhanced by insolation [15] , [19] , the wider troughs of the Sr/Ca variability likely represent, and thus are assigned, to daytime calcification. The narrower peaks are assigned to night time. This assignment effectively aligns Sr/Ca variability with insolation variability, which drives water-temperature variability. However, because the heat capacity of water is high, water temperature is not able to respond immediately to insolation changes. Therefore, insolation variability leads temperature variability ( Fig. 2b,c ). Consequently, Sr/Ca has a negative correlation with insolation but no correlation with temperature ( Supplementary Fig. S5a,b ). The lack of a relationship with temperature is a direct consequence of the age model adopted in this work, and it is quite possible that temperature has significant impact on Sr/Ca, especially given that temperature is the major determinant in oxygen isotopic ratios of a giant clam [15] . However, available reports of Sr/Ca measurements on bivalve shells suggest no temperature control [20] , [21] . Also, a decreasing trend of water temperature observed from 1–13 October ( Fig. 2c ) has no corresponding trend in the Sr/Ca data ( Fig. 2a ), suggesting that temperature may not be the principal driver of Sr/Ca. Because of the ambiguity in the Sr/Ca age model and the fact that insolation does not produce a smooth sinusoidal curve, it is not fruitful to carry out phase analysis to determine precise lead/lag relationships between Sr/Ca and environmental variables shown in Fig. 2 , which includes insolation, temperature, sea level, and precipitation. Instead, a simple autocorrelation analysis of these variables, except for precipitation that is episodic, is presented ( Supplementary Fig. S6 ). It shows a periodic variation in the Sr/Ca ratio over a 20-μm shell distance, which likely represents mean daily growth bandwidth and a single day. Insolation and water temperature have an obvious 24 h cycle, whereas tidally driven semidiurnal sea level change has an ~12 h cycle. Tidal forcing is therefore not likely the principal controller of Sr/Ca variation in this work, even though there appear to be tidal modulations of Sr/Ca in a Pacific reef coral [22] . The way by which the daily light cycle was assigned to Sr/Ca variability in this study has implications on consideration of the geochemical driving mechanism of the Sr/Ca variability. The incorporation of Ca and Sr into the calcite skeleton from ambient sea water occurs in two steps: first, ionic transport from ambient sea water to extrapallial fluid (EPF); and second, precipitation from EPF to shell skeleton. Elemental fractionation that acts on these steps can cause variability in Sr/Ca ratio in aragonite skeleton. In the first step, two mechanisms have been hypothesized to cause Sr/Ca fractionation in bivalve shells [20] , [21] . They are the Ca-ATPase hypothesis and the Ca-channel hypothesis. According to the Ca-ATPase hypothesis, selective incorporation of Ca is expected at high-calcification rates, induced by enzymes activated by solar energy. This would reduce the Sr/Ca ratio in EPF and widen the growth band during daytime. These predictions are consistent with the observations ( Fig. 1e ). In the Ca-channel hypothesis, however, a reduction of Ca selectivity is expected to occur at high calcification rates, thus leading opposite predictions inconsistent with observations. One other process in the second step, inorganic precipitation of aragonite, can cause kinetic fractionation without changing EPF compositions. It is expected to cause positive correlation between Sr/Ca and precipitation rate [23] , so that the shell Sr/Ca is predicted to increase as aragonite is preferentially precipitated from EPF during daytime. This is not supported by observations. The dominant mechanism that causes Sr/Ca variability in bivalves in this study thus appears to be the Ca-ATPase process. The high-resolution Mg/Ca and Ba/Ca data accompanying the Sr/Ca data are presented in Fig. 4 . The Mg/Ca data also appear to show a diurnal cycle, but the amplitude is rather large and highly irregular. A few reports have described a positive correlation between the Mg/Ca ratio and temperature for Mytilus trossulus [24] and Crassostrea virginica [25] , although these earlier data were obtained using a conventional analytical method. There is a slight positive correlation between the Mg/Ca ratio and seawater temperature ( Supplementary Fig. S5d ). Spike-type enrichment of Mg observed previously in coral skeletons [26] , [27] resembles the observations described in this work. The irregular spikes possibly indicate the importance of other as-yet-unidentified controls, including biological controls, on Mg/Ca. As with Sr/Ca data, Mg/Ca has no obvious correlation with precipitation or sea level (compare Figs 2d,e and 4a ). This is supported by the autocorrelation analysis of these data. There is a periodic component in Mg/Ca data ( Supplementary Fig. S6a ), whereas the precipitation is episodic. The Ba/Ca data show large amplitude variability but no obvious diurnal cycle. Ba/Ca variation may be attributable to changes in precipitation, because Ba/Ca is apparently affected by reef nutrient contents [28] , [29] , which are occasionally influenced by river water. Among these high-resolution record of Ba/Ca, Sr/Ca and Mg/Ca ratios, there is no obvious correlation except for Sr/Ca and Mg/Ca ratios (both have a periodic component). This is in contrast to observed, synchronous variations in these ratios in corals that have been attributed to changes in ambient water temperature [30] . This may be partly due to the stronger biological control in a giant clam than in corals. This work presented new measurements of Sr/Ca, Mg/Ca and Ba/Ca in the finest temporal resolution to date in the carbonate geochemistry literature [1] , [2] , [3] , [4] , [5] , [6] , [7] , [8] , [9] . Although there is some ambiguity in the age model, the giant clam Sr/Ca data clearly demonstrated the daily light cycle, which we attributed to insolation-driven, differential rates of growth and calcification. This attribution is preliminary at this time, as it is not possible to quantify other possible controls. This includes enhanced growth rates due to increased availability of nutrients or higher temperatures. Because of the regular diurnal cycle, the temperature effect in particular is a real possibility, especially as its effect on the oxygen isotope composition of carbonate shells is well documented [15] . To realize the possibility of developing the giant clam Sr/Ca as a useful proxy of insolation or some other aspect of the daily light cycle, it will be necessary to establish the age model with more confidence and isolate the effects of temperate and insolation. Analysis of δ 18 O at the same 2 μm resolution with a 0.1‰ error as the Sr/Ca data in this work would make a significant contribution to this effort, but such analysis would be difficult given present experimental techniques. Instead, cultivation of the giant clam under different, controlled environmental settings may be more feasible. For example, cultivation at a constant temperature with ambient light can isolate the temperature control on the Sr/Ca ratio. Still easier may be controlling for light with a simple cover to shield light reaching the giant clam. Another method may be to expose the giant clam to a dye, possibly a Sr isotope spike (enriched 87 Sr), at particular times of the day to make the times, so that the peaks and troughs of the Sr/Ca variation can be definitively assigned to night and day. These are imminently feasible and point the way forward in realizing the exciting possibility of developing a high-resolution daily light cycle proxy. NanoSIMS analyses Mounted samples were polished with a polishing sheet with fine alumina grains embedded on the surface. Final polishing was done with a 1-μm alumina suspension. The polished surface was coated with Pt-Pd to avoid charging during the analysis. Measurement of major and trace elements was performed by a NanoSIMS installed at the Atmosphere and Ocean Research Institute, the University of Tokyo. There are two types of measurements; high- and low-resolution analysis. For the high resolution, a ~100-pA primary beam of 16 O − was focused, ~2 μm spot in diameter. For the low resolution, an ~10-nA primary beam with 10 μm spot was used. Secondary ions were extracted by an accelerating voltage of 8 kV, introduced into a Mattauch–Herzog geometry, and 24 Mg, 44 Ca, 88 Sr and 138 Ba ion were measured simultaneously by multi-collector system. Molecular interference was not observed except for 40 Ca 2 26 Mg 16 O 2 on 138 Ba peak. The 138 Ba/ 44 Ca ratio was corrected based on the observed 24 Mg/ 44 Ca ratio and the estimated 40 Ca 2 26 Mg 16 O 2 / 24 Mg ratio [17] . All data were calibrated against a natural calcite rock from Mexico, which is homogeneous for the Mg/Ca and Sr/Ca ratios [31] , [32] . ICP-MS analyses To check the validity of low-resolution data, the Sr/Ca and Mg/Ca ratios of the sample with a similar trajectory (see C–D in Supplementary Fig. S2a ) parallel to the NanoSIMS analysis (A–B) were measured by ICP-MS. The clam shell was sampled by a micro-drilling machine, making a spot of about 1 mm diameter and 1 mm deep with 1.5 mm interval. Scraped powder was dissolved by HNO 3 and prepared for the analysis. Intensities of 9 Be, 24 Mg, 43 Ca, 45 Sc, 48 Ca, 88 Sr, 137 Ba and 209 Bi were measured by ICP-MS where 9 Be, 45 Sc and 209 Bi were the internal standard elements added into the sample solution. Observed 24 Mg/ 43 Ca, 88 Sr/ 43 Ca and 137 Ba/ 43 Ca ratios were calibrated against those of a standard sample (JCt-1) prepared and distributed by National Institute of Advanced Industrial Science and Technology, AIST in Japan. Both Mg/Ca and Sr/Ca ratios are shown in Supplementary Fig. S2b and S2c , respectively, where the NanoSIMS data are given by count ratios. There is an overall agreement, suggesting that the low-resolution data of the NanoSIMS are reliable and assured by the ICP-MS data. Duplicate and high-resolution data To assess the fidelity of the diurnal variation of Sr/Ca presented in Fig. 2 , we have duplicated the experiment using another giant clam shell cultivated at the same location (Kabira coral reef) and time (from 27 March 2002 to 14 October 2005). Analytical conditions are the same as the first high-resolution data set using a 2-μm spot with a 2-μm interval at the inner edge. Variations of Sr/Ca, Mg/Ca and Ba/Ca ratios are shown in Supplementary Fig. S1 . There is significant diurnal variation of Sr/Ca, which is clearly responding to the daily light cycle. It is possible to layer-count the dates, even though the morning data of the collection data are missing. The number of data in a single day is 5–7, smaller than that of the first data set, which had about 11 data. As the experiment was precisely conducted with a 2-μm interval, the daily bandwidth of this sample is smaller than that of Fig. 2 . This suggests that the growth rate is variable among the individuals, even under the same environmental conditions. The Sr/Ca ratios of 7 October are apparently irregular, consistent with the lowest insolation during the day ( Fig. 2b ). On the basis of the age model of the new data in Fig. 2 , there is a slight positive correlation between the Sr/Ca and Mg/Ca ratios. No diurnal cycle is observed in the Ba/Ca ratio. Autocorrelation of high-resolution record and environmental conditions Supplementary Fig. S6 shows the autocorrelation analysis of Mg/Ca ratio, Sr/Ca ratio, insolation, water temperature and sea level derived from the high-resolution data presented in Fig. 2 . Precipitation is not considered, because there is no periodic component to it. The horizontal axis of the Mg/Ca and Sr/Ca ratios is based on shell distance from the inner edge in micrometre, whereas the unit of meteorological parameters is in hour. There are apparent periodic variations of Mg/Ca and Sr/Ca ratios with a 20-μm interval. On the other hand, the cycle is 24 h for the insolation and water temperature, whereas it is 12 h for the sea level. There are two peaks per day in sea level variation between September 30 and October 8, while only one broad peak is seen between 25 and 28 September ( Fig. 2d ). These temporal variations are significantly different from those of Ma/Ca and Sr/Ca, which has generally one peak per day ( Fig. 4a ), suggesting that tidal forcing is not the principal control in this work, even though there are tidal modulations of Sr/Ca ratios in a Pacific reef coral. Relation of Sr/Ca and Mg/Ca to insolation and temperature On the basis of the assigned timing of the long, low-resolution Sr/Ca ratio data relative to meteorological data shown in Fig. 3 , there is a slight negative correlation between monthly mean daily insolation and the corresponding monthly mean Sr/Ca ratio ( Supplementary Fig. S3a ) but no relation between seawater temperature and the Sr/Ca ratio ( Supplementary Fig. S3b ). The relationship between insolation and Sr/Ca ratio is approximated by a method for linear curve fitting with both variables in error (York method) as where P1 denotes the daily insolation with the unit of MJ m −2 . Errors assigned to the slope and intercept are 1 σ . The relationship may imply that the insolation control on the Sr/Ca ratio is negative. If the same quantitative relation is sought for the high-resolution record shown in Fig. 2 , the equations would be: where P2 denotes the hourly insolation with the unit of MJ m −2 and the fitting was made based on the both variable in error and the correlation coefficient is 0.230. This relation was derived with 3-point averaged, daily peak values for Sr/Ca and insolation. It ignored the apparent outlier of the October 7 value ( Supplementary Fig. S5a ). There is no apparent relationship between the Sr/Ca and temperature with the correlation coefficient of 0.004 ( Supplementary Fig. S5b ). Similar average of daily peak values for Mg/Ca was calculated and plotted against the insolation ( Supplementary Fig. S5c ) and temperature ( Supplementary Fig. S5d ). There is a positive correlation between the Mg/Ca and temperature with the correlation coefficient of 0.465. Low resolution Mg/Ca and Ba/Ca data The NanoSIMS low resolution Sr/Ca data are confirmed by ICP-MS ( Supplementary Fig. S2 ). The NanoSIMS Mg/Ca and Ba/Ca ratios of low-resolution data are shown in Supplementary Fig. S4 . Experimental errors are 1.5% (1 σ ) for Mg/Ca ratios and 5% (1 σ ) for Ba/Ca ratios, estimated by repeated measurements of the standard calcite. In contrast to the Sr/Ca ratio, the Mg/Ca ratio has weak negative correlations with both the monthly mean surface seawater temperature and insolation. On the other hand, the Ba/Ca ratio has no relation with temperature but a positive correlation to insolation. Select intervals and uncertainty in age model in high-resolution data The long, low-resolution Sr/Ca data presented in Fig. 3 is examined in greater detail in four short segments at select intervals ( Supplementary Fig. S7 ). The intervals are at distances of 1,000–1,050, 2,000–2,050, 3,000–3,050, and 4,000–4,050 μm from the inner edge. Shown are Sr/Ca and insolation, water temperature, and precipitation at estimated dates. There are two problematic aspects to the estimated dates or the age model of this long record. First, a 10% reduction in the length of the calendar year, as determined by layer counting the Sr map bands ( Fig. 1e ), was necessary to bring about an overall match in the seasonal variations in Sr/Ca and insolation. As a result, there are four Sr/Ca peaks during two very cloudy (<0.5 MJ m −2 ) and rainy days during 22–24 March period ( Supplementary Fig. S7a .) For unexplained reasons, it seems Sr/Ca variations do not faithfully reflect the daily light cycle on cloudy days. Without assigning double enrichment bands per day on cloudy days, the year 2004, for example, with 38 cloudy days (<5 MJ m −2 at Ishigaki Island) would have been overestimated by 10%. The Sr/Ca data presented in Fig. 3 include this 10% adjustment in lining it against meteorological data. Anyway there is a relationship between the amplitude of Sr/Ca variation and insolation in a day. When we take three-point average of the peak and trough of Sr/Ca ratios and the insolation peak for an individual day in Supplementary Fig. S7 , there is a positive relation between the insolation peak and the difference of Sr/Ca ratios from the peak to trough with a correlation coefficient of 0.848. A similar relationship is observed between the water temperature and the Sr/Ca ratio with the coefficient of 0.935. These data suggests that the Sr/Ca ratio may be a proxy the insolation. The second problematic aspect of our age model is the length of the Sr/Ca record represents ~2 years of calcification, while the entire duration of the giant clam cultivation (27 March 2002 until 14 October 2005) is one-and-half years longer. The starting time of calcification (mid-September 2003) was estimated by counting backwards from the inner edge, which is assumed to have been calcified on the day of collection. This may be due to that the young and juvenile portion of the shell was lost by cutting and grinding processes for making the sample cross section. Another possibility is that the giant clam did not calcify during the first year and half, which seems quite long even after considering the fact that very young and juvenile stages of the giant clam likely did not calcify in any significant manner. Resolving this puzzle is an issue to be addressed in the future, perhaps by marking the times of calcification with enriched isotope tracers. How to cite this article : Sano, Y. et al . Past daily light cycle recorded in strontium/calcium ratios of giant clam shell. Nat. Commun . 3:761 doi: 10.1038/ncomms1763 (2012).